A hybrid high-speed atomic force–optical microscope for visualizing single membrane proteins on eukaryotic cells High-speed atomic force microscopy is a powerful tool for studying structure and dynamics of proteins. So far, however, high-speed atomic force microscopy was restricted to well-controlled molecular systems of purified proteins. Here we integrate an optical microscopy path into high-speed atomic force microscopy, allowing bright field and fluorescence microscopy, without loss of high-speed atomic force microscopy performance. This hybrid high-speed atomic force microscopy/optical microscopy setup allows positioning of the high-speed atomic force microscopy tip with high spatial precision on an optically identified zone of interest on cells. We present movies at 960 ms per frame displaying aquaporin-0 array and single molecule dynamics in the plasma membrane of intact eye lens cells. This hybrid setup allows high-speed atomic force microscopy imaging on cells about 1,000 times faster than conventional atomic force microscopy/optical microscopy setups, and allows first time visualization of unlabelled membrane proteins on a eukaryotic cell under physiological conditions. This development advances high-speed atomic force microscopy from molecular to cell biology to analyse cellular processes at the membrane such as signalling, infection, transport and diffusion. High-speed atomic force microscopy (HS-AFM) [1] has been proven to be a unique and powerful tool for the concomitant analysis of the structure and dynamics of single biomolecules [2] . HS-AFM was used to visualize myosin-V walking [3] , cellulase cellulose degradation [4] , F 1 -ATPase rotary catalysis [5] , bacteriorhodopsin photocycle [6] , and OmpF diffusion and interaction [7] . However, HS-AFM has been restricted so far to well-controlled molecular systems of purified proteins under well-controlled conditions. These systems were characterized by a limited number of pure molecular species with small corrugation, mainly because the fast z-piezo that follows the topography profile has a small extension range (typically 400 nm; ref. 8 ). Recently, the development of a wide-range HS-AFM scanner allowed the first nanoscale observation of molecular movements at two frames per second on living bacteria [9] . Historically, AFM debuted as early as 1990 for cell imaging applications [10] , prompted by the need to perform cell structural analysis at a resolution superior to light microscopy. However, AFM images of cells revealed rather the cell interior, like actin filaments, than the membrane structure of the cells. Later, AFM and optical microscopy (OM) were combined in order to take advantage of OM’s large-scale overview imaging capacities and its power to analyse fluorescence signal targets of proteins of interest [11] . For this purpose, AFMs were built in a table-top configuration and mounted on inverted optical microscopes [12] . In order to avoid modifications of the conventional inverted OM, two types of table-top AFM configurations were built. In one of them, the AFM tip and the scanner is combined into a single moving component, and in the other a large optical microscope sample stage on which the AFM sample is mounted needs to be moved. In both cases, there is a loss of AFM performance. In the tip-scanner configuration, the laser detection must be coupled to the moving cantilever, while for the second case, the sample stage that needs to be moved is complex and heavy. Both types of structures are prone to capture environmental noise and feature innate resonance frequencies. Furthermore, massive objects do not allow sub-millisecond mechanical response, thus precluding individual protein imaging at high resolution and high speed. In this work, we integrate an OM path into our HS-AFM, maintaining the structure of the HS-AFM setup [1] , and hence not compromising HS-AFM performance in terms of speed and resolution. To achieve this, we choose a completely different approach compared with most (if not all) AFM/OM integration developments: instead of building a table-top AFM mountable on an inverted optical microscope, accepting loss of AFM performance, we build an optical path into our HS-AFM setup, accepting minimal trade-offs in OM performance. We show that our setup can acquire bright field and fluorescence OM images of biological samples, and that it allows HS-AFM tip positioning with high precision guided by OM. Finally, we show that it achieves HS-AFM imaging of individual membrane proteins on eukaryotic cells and record their dynamics at an imaging rate of 960 ms per frame. This accomplishment opens the door to a wide range of real-time studies of molecular dynamics in membrane processes on living cells. Development of hybrid HS-AFM and fluorescence microscope In order to integrate an OM path into the HS-AFM ( Fig. 1 and Fig. 2a ), we added and exchanged several elements to and from the HS-AFM setup, previously designed by Ando et al [1] . The original laser diode of the HS-AFM system that reads the cantilever position was changed to a far-red superluminescent diode (SLD) with 750 nm wavelength and low coherence ( Fig. 1 , label 1). The use of the SLD 750 nm allowed the optical separation of the AFM cantilever detection ( Fig. 1 , red arrows) from the visible light OM signals (as will be detailed below). We removed the λ /4 plate and the polarization beam splitter in the optical path that was initially designed to separate the incident and the reflected laser beams to and from the cantilever, respectively. The polarization beam splitter has been replaced by a 45° mirror that deflects only the reflected laser beam. Indeed, we physically separated the incident and the reflected laser beams by about 1 mm by displacing the incident laser by 0.5 mm with respect to the centre position of the objective that focuses the laser onto the backside of the cantilever. The mirror directs the entire reflected laser beam onto the photo detector split diode, while the beam splitter did not reflect all the light and part of the beam was transmitted into the SLD potentially creating optical feedback. This alteration resulted in a higher signal-to-noise ratio and hence more sensitivity of the deflection detection. Further major changes/integrations to build the OM path are the following: in the heart of the setup, we integrated a low-pass (<700 nm) dichroic mirror ( Fig. 1 , label 4), allowing recovery of the AFM SLD 750 nm beam and the passage of optical signals below 700 nm; a fluorescence light source ( Fig. 1 , label 2) injects light through a fluorescence filters cube ( Fig. 1 , label 6) that allows the tuning of the wavelength of the incident light for excitation of the sample-specific fluorophore ( Fig. 1 , blue arrow). The fluorescence filters cube is identical to the ones used in conventional fluorescence microscopes and allows the same versatility for fluorescence experiments. The cube is located outside of the hard body of the HS-AFM allowing easy exchange of the filters for the fluorophore excitation wavelength needed ( Fig. 2a ). The reflected light with the emission wavelength of the fluorophore ( Fig. 1 , green arrow) is filtered again in the fluorescence filter cube ( Fig. 1 , label 6) to be recorded exclusively and with low background noise on a CCD camera ( Fig. 1 , label 7). A large-area visualization camera is used to align the laser on the tip and place the sample holder over the tip for easy tip engagement ( Fig. 1 , yellow arrows). The switching between the laser alignment camera exit located further down in the optical path than the fluorescence or bright field CCD camera light recovery pathway is done with an optical switch 45° mirror ( Fig. 1 , dashed outline) that can be controlled with a linear motor stage. Finally, for bright field OM, we inject light ( Fig. 1 , label 3) from the side into a specially designed novel sample support—a cube composed of two aluminum-coated prisms of 1.5-mm edge length ( Fig. 1 , label 5; Fig. 2c ). The bright field light is transmitted through a thin (<100 μm) mica sample support—like a light table—and is finally recorded on the CCD camera ( Fig. 1 , white arrows). All light is funneled into and out of the sample chamber through the same objective [1] . The physical uncoupling of the light sources and the CCD camera ( Fig. 1 , elements shaded in light blue) from the HS-AFM main body prevents transfer of mechanical destabilizations, such as vibrational noise, from these elements to the HS-AFM. This HS-AFM/OM hybrid has uncompromised HS-AFM imaging performance. 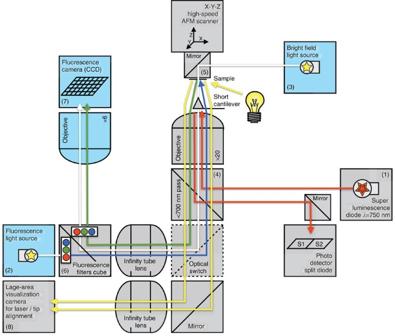Figure 1: Schematic of the integrated HS-AFM–OM hybrid setup. The essential elements integrated are: a 750 nm SLD for cantilever position detection (1), two light microscopy sources (2 and 3), a 700-nm low-pass beam splitter (4), a miniaturized mirror sample support (5), a fluorescence filter cube beam splitter (6) and a high-resolution CCD camera (7). A large-area visualization camera allows the alignment of the laser on the HS-AFM tip (8). Several elements (blue) are physically uncoupled from the HS-AFM body (grey). Figure 1: Schematic of the integrated HS-AFM–OM hybrid setup. The essential elements integrated are: a 750 nm SLD for cantilever position detection (1), two light microscopy sources (2 and 3), a 700-nm low-pass beam splitter (4), a miniaturized mirror sample support (5), a fluorescence filter cube beam splitter (6) and a high-resolution CCD camera (7). A large-area visualization camera allows the alignment of the laser on the HS-AFM tip (8). Several elements (blue) are physically uncoupled from the HS-AFM body (grey). 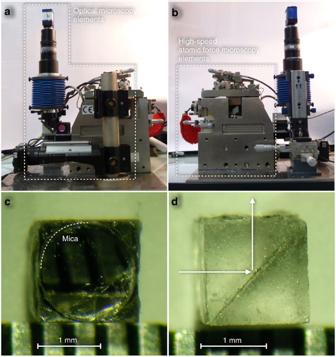Figure 2: Integrated HS-AFM–OM hybrid setup and the miniaturized mirror sample support. (a) Side view roughly corresponding to the schematic inFig. 1. The elements of the OM pathway are outlined. The bright field light source incident stage is facing the viewer, in the schematic it is depicted to the HS-AFM long axis. (b) Side view from the opposite side to (a). The elements of the HS-AFM are outlined. Some of the elements (for example, light sources) that are linked over cables to the dark box/Faraday cage, of which the setup had to be taken out, are not present in the photographs. (c) Top view: the 45° mirror glass cube sample holder for lateral light injection has dimensions of 1.5 mm × 1.5 mm × 1.5 mm. On its surface a 1.5-mm-diameter mica disk is glued with a transparent glue. Through the mirror cube the 0.5-mm scale lines of the rule can be seen, illustrating the function for lateral light injection (scale bar: 1 mm). (d) Side view: the 45° mirror glass cube is composed of two aluminum-coated glass prisms glued to each other. The interface between the two elements is visible as a diagonal line from the side. The white arrows illustrate the bright field light source injection and exit through the mica sample support (scale bar: 1 mm). Full size image Figure 2: Integrated HS-AFM–OM hybrid setup and the miniaturized mirror sample support. ( a ) Side view roughly corresponding to the schematic in Fig. 1 . The elements of the OM pathway are outlined. The bright field light source incident stage is facing the viewer, in the schematic it is depicted to the HS-AFM long axis. ( b ) Side view from the opposite side to ( a ). The elements of the HS-AFM are outlined. Some of the elements (for example, light sources) that are linked over cables to the dark box/Faraday cage, of which the setup had to be taken out, are not present in the photographs. ( c ) Top view: the 45° mirror glass cube sample holder for lateral light injection has dimensions of 1.5 mm × 1.5 mm × 1.5 mm. On its surface a 1.5-mm-diameter mica disk is glued with a transparent glue. Through the mirror cube the 0.5-mm scale lines of the rule can be seen, illustrating the function for lateral light injection (scale bar: 1 mm). ( d ) Side view: the 45° mirror glass cube is composed of two aluminum-coated glass prisms glued to each other. The interface between the two elements is visible as a diagonal line from the side. The white arrows illustrate the bright field light source injection and exit through the mica sample support (scale bar: 1 mm). Full size image HS-AFM imaging of cells guided by OM The HS-AFM/OM hybrid setup was operated with short cantilevers ( Fig. 3a ), 6 μm long, 2 μm wide and 100 nm thick, with a high aspect ratio tip centred at its end ( Fig. 3a , inset). These cantilevers are identical to those used for molecular HS-AFM imaging [7] . In bright field OM, the cantilever appears as a black bar ( Fig. 3b , left). Two-dimensional cross correlation of the bright field image of the cantilever with a computed black circle of 2 μm diameter ( Fig. 3b , inset) results in a cross-correlation map, in which the tip localization is characterized by a cross-correlation value maximum ( Fig. 3b , right). This rapid procedure allows determination of the lateral tip position with a precision better than 100 nm. Once the relative position of the HS-AFM tip is defined, it can be placed on cells guided by bright field ( Fig. 3c ) or fluorescence ( Fig. 3d ) OM. Although the cantilever is mainly visible in bright field mode rather than in fluorescence microscopy mode, knowledge of the localization of the tip, defined by the above described cross-correlation procedure, allows its placement on a fluorescent zone of interest. 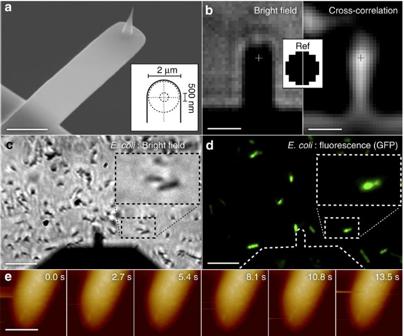Figure 3: Placement of HS-AFM tip and HS-AFM–OM overview imaging ofE. colicells. (a) Scanning electron microscopy image of a HS-AFM cantilever with 6 μm length, 2 μm width and 0.1 μm thickness. Inset: geometrical characteristics of the HS-AFM cantilever apex (scale bar: 2 μm). (b) Bright field microscopy image of the cantilever (left) and corresponding cross-correlation map (right) after cross-correlation with a computed disk of diameter 2 μm (inset). The cross in the cross-correlation map identifies the calculated tip localization (scale bars: 2.5 μm). (c) Bright field, and (d) fluorescence (GFP expression) OM images ofE. colicells in the HS-AFM/OM setup (scale bars: 10 μm). (e) HS-AFM overview image series on anE. colicell, selected by the positive fluorescence signal, see (d) (scale bar: 1 μm). Figure 3: Placement of HS-AFM tip and HS-AFM–OM overview imaging of E. coli cells. ( a ) Scanning electron microscopy image of a HS-AFM cantilever with 6 μm length, 2 μm width and 0.1 μm thickness. Inset: geometrical characteristics of the HS-AFM cantilever apex (scale bar: 2 μm). ( b ) Bright field microscopy image of the cantilever (left) and corresponding cross-correlation map (right) after cross-correlation with a computed disk of diameter 2 μm (inset). The cross in the cross-correlation map identifies the calculated tip localization (scale bars: 2.5 μm). ( c ) Bright field, and ( d ) fluorescence (GFP expression) OM images of E. coli cells in the HS-AFM/OM setup (scale bars: 10 μm). ( e ) HS-AFM overview image series on an E. coli cell, selected by the positive fluorescence signal, see ( d ) (scale bar: 1 μm). Full size image The benefit provided by implementing both bright field and fluorescence OM modes and the possibility to switch between these can be illustrated on Escherichia coli cells transformed with an overexpression plasmid for green fluorescence protein (GFP) production. Some of the E. coli cells grown to stationary phase and without antibiotic selection express GFP, while others do not fluoresce, offspring from cell divisions with loss of the GFP expression plasmid in one daughter cell. Therefore, as a proof of concept, many more bacteria are visible in bright field mode ( Fig. 3c ) than in fluorescence microscopy ( Fig. 3d ). For example, of two neighbouring E. coli cells visualized in bright field mode ( Fig. 3c , inset), only one is fluorescent and therefore visible when detecting GFP only ( Fig. 3d , inset). This conceptual demonstration shows the power of the fluorescence OM integration allowing the HS-AFM analysis to be directed towards a molecule or cell, or a subregion of a cell of interest. Consequently, dynamic HS-AFM imaging can be acquired on a specifically chosen E. coli cell ( Fig. 3e ; Supplementary Movie 1 ). The HS-AFM/OM hybrid setup allows therefore the HS-AFM tip to be placed on the surface of a cell with certain characteristics, that is, the expression of a particular molecule that can be identified by the co-expression of a fluorescence tag. This particular feature opens a wide range of novel applications to HS-AFM, making it a powerful tool for cell biology. Moving on from prokaryotic E. coli cells, we investigated the architecture of mammalian eye lens junctional microdomains at high spatial and temporal resolution. Junctional microdomains are mainly constituted of lens-specific AQP0 that are thought to fulfill a double function as water channels [13] and cell adhesion molecules [14] . While junctional AQP0 has been described by early freeze fracture electron microscopy [15] , at high resolution after reconstitution by electron crystallography [14] and in isolated lens membranes by AFM [16] , [17] , [18] , they have not been observed on native cells in physiological buffer. Beyond structural aspects, questions remain unanswered concerning the dynamics of junctional microdomains, notably in the context of assuring cell adhesion during tissue deformation upon lens accommodation (focusing to different distances). Following placement of the HS-AFM tip on the lens cell surface ( Fig. 4a ), overview HS-AFM imaging can be performed revealing the lens cell superstructure ( Fig. 4c ). Such image series visualized protruding membrane structures characteristic for fibre lens cells, prior identified by freeze fracture electron microscopy of lens tissue as the interlocking ball-and-sockets structures accommodating adhesive membrane proteins in connexin gap junctions and AQP0 thin junctions [19] ( Fig. 4c , arrow; Supplementary Movie 2 ). It has been proposed that these sockets intercalate the lens cells maintaining stability between fibre cells during visual accommodation of the lens tissue. Furthermore, short-range surface topographical features are visualized on the cell surface ( Fig. 4c ; Supplementary Movie 3 ). These corrugations have been observed by scanning electron microscopy but elude visualization under native conditions in light microscopy because of their 100–300 nm dimensions [19] . 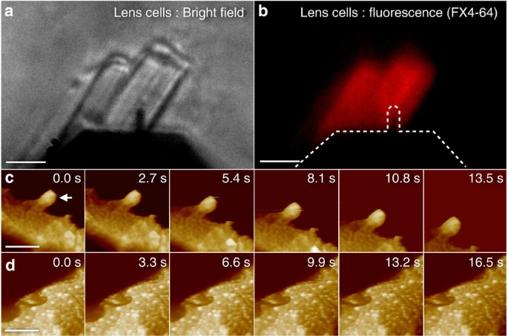Figure 4: Overview HS-AFM–OM analysis of native lens cells. (a) Bright field and (b) fluorescence (FX4-64 membrane staining) OM images of short HS-AFM cantilever placed on lens cells in the HS-AFM setup (scale bars: 10 μm). (c) and (d) HS-AFM overview image series on lens cells. Characteristic ball-and-socket structures (arrow inc) and surface hump and valley structures on the cell surfaces are identified at high resolution (scale bars: 2 μm). Figure 4: Overview HS-AFM–OM analysis of native lens cells. ( a ) Bright field and ( b ) fluorescence (FX4-64 membrane staining) OM images of short HS-AFM cantilever placed on lens cells in the HS-AFM setup (scale bars: 10 μm). ( c ) and ( d ) HS-AFM overview image series on lens cells. Characteristic ball-and-socket structures (arrow in c ) and surface hump and valley structures on the cell surfaces are identified at high resolution (scale bars: 2 μm). Full size image Importantly, we were able to detect single AQP0 on lens cells using our HS-AFM/OM hybrid setup. To the best of our knowledge, this is the first time that unlabelled single membrane proteins on a eukaryotic cell are visualized under physiological conditions. This was possible owing to minimal tip–sample interaction using small oscillation free amplitudes, minimal free-amplitude damping as setpoint and a high cantilever resonance frequency. Under such conditions, the sample was subjected to very low impulses I of ~10 aN s (attonewton times second), following [20] , , where k c is the spring constant of 0.1 N m −1 , Q is the quality factor of the cantilever in liquid of 1, A is the imaging amplitude, that is, 0.9 times the free amplitude A 0 of 2 nm, and the contact time t is defined as 10% of the oscillation period T that is the inverse of the resonance frequency of 600 kHz. For comparison, in conventional AFM setups, the impulse is about three orders of magnitude higher. We can identify AQP0 by the characteristic square array packing in lens cells, previously described by freeze fracture electron microscopy [15] and by AFM of isolated membranes [16] , [17] , [18] , with packing parameters of a = b =6.5 nm, γ =90° ( Fig. 5a ). Importantly, association and dissociation dynamics of AQP0 to and from the array can be observed at a frame rate of 960 ms ( Fig. 5a arrow heads; Supplementary Movie 4 ), emphasizing the strong potential of HS-AFM imaging for the analysis of the structure and dynamics of membrane processes with our novel hybrid setup. The AQP0 array itself displayed mobility on the lens cell surface as revealed by cross-correlation-based tracking ( Fig. 5b ). The trace is non-directional with varying displacement distances in consecutive frames typical for normal diffusion. Displacement distance histogram analysis ( Fig. 5c ) and root mean square displacement (RMSD) analysis ( Fig. 5d ) of the diffusion corroborate this finding. The displacement histogram is described by a Gaussian distribution function with a peak at 1.5 nm between successive frames (time interval 960 ms). The RMSD displacement, following the power law: σ ( r ) 2 ~ Dt α (σ is the mean displacement, D is the diffusion constant and t the lag time), results in a value α =0.94, characteristic of Brownian diffusion, discarding active cellular processes or piezo drift (that follows a directional trend during relaxation [21] ). Liberty of free diffusion of the AQP0 arrays allows the junctional microdomains to account for stress between cells during tissue shape changes. Furthermore the junctional microdomains are in a dynamic equilibrium with single AQP0 associating and dissociating providing further potential for adaptation. 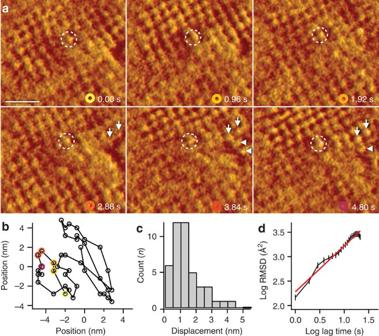Figure 5: HS-AFM analysis of unlabelled AQP0 on a lens cell under ambient conditions. (a) HS-AFM image series (960 ms frame rate) showing the typical square AQP0 lattice (a=b=6.5 nm,γ=90°) and AQP0 assembly dynamics (see arrow heads in images 3.84 and 4.80 s) neighbouring stable AQP0 molecules (arrows). A strongly protruding molecule (dashed circle) and its molecular environment have been used to analyse the displacement of the array (scale bar: 20 nm). (b) Tracking trace of the AQP0 array (the relative position of the array in the first six frames is highlighted by coloured circular markers). (c) Displacement distance histogram and (d) RMSD plot of (b) with vertical bars indicating the s.d.’s of the data points and least square linear fit determining the slopeα=0.94 (red line;R2=0.97). Figure 5: HS-AFM analysis of unlabelled AQP0 on a lens cell under ambient conditions. ( a ) HS-AFM image series (960 ms frame rate) showing the typical square AQP0 lattice (a=b=6.5 nm, γ =90°) and AQP0 assembly dynamics (see arrow heads in images 3.84 and 4.80 s) neighbouring stable AQP0 molecules (arrows). A strongly protruding molecule (dashed circle) and its molecular environment have been used to analyse the displacement of the array (scale bar: 20 nm). ( b ) Tracking trace of the AQP0 array (the relative position of the array in the first six frames is highlighted by coloured circular markers). ( c ) Displacement distance histogram and ( d ) RMSD plot of ( b ) with vertical bars indicating the s.d.’s of the data points and least square linear fit determining the slope α =0.94 (red line; R 2 =0.97). Full size image This first analysis of dynamic membrane protein imaging on a eukaryotic cell opens the field for analyses of degrees of order and organization in cytoplasmic membranes, especially in the context of current controversial questions concerning the mosaic structure [22] and the segregation of membrane constituents into functional domains/rafts [23] . In the last 20 years, a paradigm shift has emerged in cell biology: the plasma membrane is not a random two-dimensional fluid of lipids with floating membrane proteins [24] , but rather a complex mosaic of spatially segregated structural and functional entities composed of membrane proteins, lipids and sugars [22] . This novel concept is the result of data from several indirect techniques, lead by soft membrane extractions combined with gel electrophoresis and light microscopy [23] , [25] , [26] , [27] . Visualization of native membrane proteins directly on eukaryotic cells in physiological environments is an important step towards understanding membrane processes, such as signalling and transport, but owing to technological difficulties this has not been possible in the past. Here, we have presented images of AQP0 on lens fibre cells immersed in physiological buffer and at ambient temperature and pressure ( Fig. 5a ). To achieve this, we developed an integrated HS-AFM/OM hybrid setup that allows placement of the short HS-AFM cantilever on areas of interest on a cell, providing the first image series of membrane protein association and dynamics on a eukaryotic cell. AQP0 arrays display slow but free Brownian diffusion. This possibility of free displacement of the junctional microdomains has importance in the context of the tissue integrity during lens accommodation. Indeed, lens cell must maintain tight contacts while undergoing lateral rearrangement when the lens changes its shape. Free diffusive adhesion platforms represented by junctional AQP0 arrays can comply for adhesion within a flexible tissue. Recently, the architecture and dynamics of AQP4 orthogonal arrays have been analysed by OM [28] . While the action of AQP4 as an adhesion molecule is still debated [28] , the characteristics of AQP4 and AQP0 arrays compare well. Both proteins form regular arrays slightly smaller than the diffraction limit of light with various reorganization events as a function of time. The arrays of both AQP4 and AQP0 reveal slow Brownian motion. Here, we find for AQP0 arrays a diffusion constant of ~5 × 10 −15 cm 2 s −1 while AQP4 arrays diffuse with ~1 × 10 −12 cm 2 s −1 , a discrepancy that might emerge from different nature of the molecules, the different nature of the cells, as well as differences in cell preparation and observation methods used. HS-AFM features an outstanding signal-to-noise ratio capable of visualizing unlabelled proteins and their interplay with each other in a membrane [7] . The presented development allows now HS-AFM operation on cells and will therefore open novel avenues for cell biology. We anticipate that using our novel HS-AFM/OM hybrid setup, we will be able to analyse dynamic assemblies of membrane proteins implicated in cellular functions, such as signalling, transport and infection processes. For instance, HS-AFM single molecule analysis of receptor clustering guided by fluorescence microscopy appears like a straight-forward application with strong biomedical potential. Development of the hybrid HS-AFM–OM setup For the integration of the OM pathway ( Fig. 2a ) into the HS-AFM ( Fig. 2b ), several optical elements needed to be changed or integrated: the conventional laser diode (emission wavelength: 670 nm) was changed to a SLD (emission wavelength: 750 nm; EXS 7505-B001, Exalos, Schlieren, Switzerland; labelled 1 in Fig. 1 ). Two light sources for the fluorescence microscopy (PhotoFluor II, Burlington, USA; labelled 2 in Fig. 1 ) and the bright field microscopy (KL2500 LED, Schott, Clichy, France; labelled 3 in Fig. 1 ) pathways were added. A short wavelength pass dichroic filter (pass: <700 nm, Edmund Optics, York, UK; labelled 4 in Fig. 1 ) and an optical switch 45° mirror (MRA25-P01, ThorLabs, Maisons-Laffitte, France) driven by a linear motor stage (DDSM100, ThorLabs) and controlled by a servo (TBD001, ThorLabs) were integrated for switching between various optical paths. The lateral light injection sample holder (labelled 5 in Fig. 1 ; Fig. 2c ) is composed of two prisms (PRK01500, Knight Optical, Herrietshame, UK) with a 100-nm aluminum-coated interface (EM SCD 500, Leica Microsystems, Wetzlar, Germany) glued together by cyanoacrylate. This support has very similar volume and weight (3.375 mm 3 , 8.5 mg) than the original cylinder sample holder (3.534 mm 3 , 8.9 mg)—the slight difference is positively compensated by the glue in between the two prisms—important for the stability and velocity of the HS-AFM system. The fluorescence filter cube (Olympus, Tokyo, Japan; labelled 6 in Fig. 1 ) allows filtering of specific wavelengths for the excitation and light recovery of fluorescent dyes (in this work were used U-MWG for FM 4-64FX and U-MWIBBP for GFP). Finally, an infinity tube lens unit (MXA20696/70g, Nikon, Tokyo, Japan), and a × 6 macrozoom lens ( × 6, f =18−108 mm/F2.5, EHD Imaging, Damme, Germany) focuses the OM signals into a CCD camera (UK1158-M-10, 1360 × 1024 pixels; EHD Imaging; labelled 7 in Fig. 1 ). HS-AFM image series were acquired with the hybrid HS-AFM/OM setup equipped with 6-μm-long cantilevers (USC-1.2, spring constant k =0.15 N m −1 and resonance frequency f (r) =1200, kHz in air; NanoWorld, Neuchâtel, Switzerland). HS-AFM was operated in amplitude modulation mode using a novel digital high-speed lock-in Amplifier (Hinstra, Transcommers, Budapest, Hungary) that analyses the amplitude and the phase of every single oscillation cycle with a Fourier method. Optimized HS-AFM electronics were used to pilot the dynamic feedback circuit. Lens cell preparation Lens cells have been prepared from sheep lens as previously described [29] . Briefly, lenses from healthy sheep 5±2 years old were obtained from UCEA INRA (Unité Commune d’Expérimentation Animale, Jouy-En-Josas, Institut National de la Recherché Agronomique, France). Enucleation occurred within 1 h of death, with lenses frozen immediately after removal from the eye by dropping them in liquid nitrogen and subsequent storage at −80 °C. All animal treatment has been conducted according to the current European and French guidelines. Lenses were thawed for about 2 h at 4 °C in dissociation buffer (10 mM Tris, pH 8.0; 5 mM EGTA; 5 mM EDTA). The equatorial diameter of lenses was ~15 mm. The absence of cataracts was verified after thawing. Eye lenses were dissected in 2 ml (per lens) of dissociation buffer. After careful capsule removal using tweezers, cortical cells were separated gently from the nucleus by flushing buffer over the lens tissue using a 1 ml pipette. The pipette flow was enough to separate the outermost ~2 mm of cortical cells. The remaining lens nucleus was continuously flushed with the pipette to obtain the innermost nucleus, ~1 mm in diameter. This was placed on the Vari-Mix shaker to obtain a uniform suspension composed of nuclear cells only. Although relatively slow, this method assures gentle and controlled separation of different layers of cells from lens tissue. Resulting cells feature native transparency and elasticity [29] . E. coli cell preparation E. coli (BL21 DE3) cells transformed to express cytoplasmic GFP were cultured in Lysogeny broth medium containing ampicillin (100 μg ml −1 ) at 37 °C until the optical density at 600 nm was 0.9. Bacterial cells were collected and centrifuged three times at 5,000 r.p.m. (2348 G) in PBS buffer and resuspended in fresh PBS. Cells continued duplication until HS-AFM analysis about 60 min after cell washing. Cell immobilization on the hybrid HS-AFM–OM sample holder A 1.5-mm-diameter mica disk was glued onto the lateral light injection sample holder ( Fig. 2c ). The thickness of the mica must be minimized in order to assure good OM performance, and was in our experiments always thinner, 100 μm. The mica disk was pretreated using 1.2 μl of 0.1% poly-l-lysine (Sigma Aldrich, St Louis, USA) solution and left to dry at room temperature. The mica was rinsed with PBS three times. Then the entire sample holder was placed in a 500 μl Eppendorf tube with the mica disk facing up. Lens cell suspension (300 μl) were pipetted into the Eppendorf tube, followed by slow centrifugation of the tube during 5 min at 300 r.p.m. (293 G) using a balancing rotor. This procedure allows efficient lens cell adsorption onto the poly- L -lysine-treated mica. For the E. coli cells this procedure is not necessary. E. coli cell solution (1.2 μl) was simply added on the poly- L -lysine pretreated mica during 60 min for physisorption. In both cases, the sample holder was rinsed three times with PBS buffer and attached to the HS-AFM scanner. All the HS-AFM/OM measurements, on both lens cells and E. coli lens, were performed in PBS buffer. Lens cells staining Lens cells membranes were stained using FM4-64FX (Invitrogen, Carlsbad, USA). About 1.2 μl of dye solution (50 μg ml −1 ) was added during 20 min onto the sample support with the attached lens cells. Following, the sample was rinsed four times with fresh PBS. The fluorescent and bright field images were observed using the HS-AFM/OM hybrid with the cube filter U-MWG (Olympus; excitation: 510–550 nm, emission: 570 nm). Data analysis Movie analysis was performed using WSxM software (Nanotec Electronica, Madrid Spain). The analysis of the AQP0 array dynamic was performed using a Java-based HS-AFM image analysis package [21] integrated in the Image-J image analysis platform. How to cite this article: Colom, A. et al. A hybrid high-speed atomic force–optical microscope for visualizing single membrane proteins on eukaryotic cells. Nat. Commun. 4:2155 doi: 10.1038/ncomms3155 (2013).